SREBP modulates the NADP+/NADPH cycle to control night sleep inDrosophila Sleep behavior is conserved throughout evolution, and sleep disturbances are a frequent comorbidity of neuropsychiatric disorders. However, the molecular basis underlying sleep dysfunctions in neurological diseases remains elusive. Using a model for neurodevelopmental disorders (NDDs), the Drosophila Cytoplasmic FMR1 interacting protein haploinsufficiency ( Cyfip 85.1/ + ), we identify a mechanism modulating sleep homeostasis. We show that increased activity of the sterol regulatory element-binding protein (SREBP) in Cyfip 85.1/ + flies induces an increase in the transcription of wakefulness-associated genes, such as the malic enzyme ( Men ), causing a disturbance in the daily NADP + /NADPH ratio oscillations and reducing sleep pressure at the night-time onset. Reduction in SREBP or Men activity in Cyfip 85.1/ + flies enhances the NADP + /NADPH ratio and rescues the sleep deficits, indicating that SREBP and Men are causative for the sleep deficits in Cyfip heterozygous flies. This work suggests modulation of the SREBP metabolic axis as a new avenue worth exploring for its therapeutic potential in sleep disorders. Sleep supports physiological well-being, and it is evolutionarily conserved from worms to humans [1] . Sleep loss leads to severe consequences such as deficits in psychomotor vigilance, attention, cognitive functions, and cellular metabolism [2] . However, the understanding of the biological functions of sleep remains a challenge [3] . Sleep is regulated by a fine-tuned interplay between the homeostatic drive and the circadian rhythm [4] , [5] . Key genes regulating circadian rhythm have been identified [6] and are conserved from flies to humans [7] , [8] . In addition, it is known that the wakefulness status leads to the accumulation of wake-dependent homeostatic factors in the brain that promote sleep, while the sleep status clears or abrogates these factors to allow the waking state [9] . Among these factors, neurotransmitters, synaptic proteins, metabolic substrates, and immune modulators have been identified [9] . However, the molecular mechanisms that mediate sleep pressure, i.e., the homeostatic system, remain elusive. Thus, identifying molecular pathways that regulate sleep need is crucial to understanding the different functions of sleep [10] . Recent evidence shows that sleep and cell metabolism are two interconnected processes modulating each other; periods of prolonged wakefulness and insufficient sleep profoundly impact the metabolome and transcriptome profiles [11] , [12] , [13] . Different studies have suggested that sleep drives the decline in synaptic activity to consolidate or strengthen particular synapses and circuitry [14] , prevents cellular damage [15] , and favors metabolic restoration and clearance within the brain [16] , [17] . Recent work has shown that the ratio of NADP + to NADPH within sleep-inducing neurons plays a role in sleep pressure in flies [18] , and that genes involved in lipid metabolism are linked to fly sleep homeostasis [19] , [20] . Therefore, sleep may act specifically as a reparative and anabolic process at the cellular level [17] , [21] , [22] . While sleep deficits are considered comorbid symptoms associated with neuropsychiatric disorders, growing evidence supports a bidirectional effect. Lack of sleep exacerbates aggression, impulsivity, repetitive behaviors, hyperactivity, anxiety, depression, and withdrawal in psychiatric patients [23] , [24] , [25] . On the other side, behavioral impairment seems to worsen sleep homeostasis [26] . Abnormal sensory processing, over-sensitivity to environmental stimuli, and increased arousal may concur to the insurgence of delayed sleep onset problems [27] . Copy number variations (CNVs) encompassing the CYFIP1 gene are associated with increased risk for several neuropsychiatric disorders such as schizophrenia (SCZ), autism spectrum disorders (ASDs), attention deficit hyperactivity disorder (ADHD), reduced cognitive dysfunction, and motor dysfunctions [28] , [29] , [30] , [31] , [32] , [33] , [34] . Notably, sleep disturbances such as insomnia or sleep problems have been reported in individuals with BP1-BP2 microdeletion/duplication harboring the CYFIP1 gene [35] , [36] , [37] . Animal models for Cyfip1 haploinsufficiency recapitulate ASD and SCZ-related behavioral deficits and neurodevelopmental alterations [38] , [39] , [40] , [41] , [42] , [43] . We have recently shown that haploinsufficiency in the Drosophila homolog of the human CYFIP1 (and CYFIP2 ) leads to associative learning deficits and dysregulation of mitochondria homeostasis and energy metabolism impinging on GABAergic neurotransmission and ultimately affecting social behaviors [30] , [43] . Drosophila melanogaster is a powerful model for dissecting the genetics and biological pathways underlying sleep behavior [44] , [45] , [46] , [47] . Sleep in Drosophila has most of the hallmarks of mammalian sleep and is associated with a higher sensory arousal threshold and a characteristic posture. In addition, the circadian and homeostatic regulation of the sleep-wake cycle is also conserved [44] , [48] . Genetic screenings and gene profiling studies in Drosophila allowed the identification of genes and pathways affecting wakefulness and sleep, highlighting the importance of cellular metabolism, protein homeostasis, synaptic excitability, and immune response [49] , [50] , [51] , [52] , [53] . Here, we show that Cyfip heterozygous ( Cyfip 85.1 /+ ) flies have decreased sleep need at night-time onset and increased SREBP activity. We observe that the transcriptomic profile of Cyfip mutant flies is enriched in genes regulating the wakefulness-associated pathways, including lipid metabolism genes such as malic enzyme ( Men ) that is regulated by the sterol element-binding protein SREBP [54] , [55] . Men is known to reduce NADP + to NADPH, and we show that Men overproduction disrupts the NADP + /NADPH ratio before sleep time. Pharmacological and genetic dampening of SREBP activity renormalizes malic enzyme activity and the NADP + /NADPH ratio, alleviating the sleep disturbances in Cyfip heterozygous flies. Taken together, our data describe a molecular and mechanistic axis impaired in neurodevelopmental conditions associated with sleep disturbances. CYFIP regulates night-time sleep The sleep pattern of Cyfip heterozygous flies (Cyfip 85.1/ + ) [56] and control flies was assessed over 24 h (Fig. 1a ) using the Drosophila activity monitoring system (Supplementary Fig. 1a ). The average sleep amount at night was significantly reduced in Cyfip 85.1 /+ compared to control flies (Fig. 1a, b ), while no change in the daytime sleep was observed (Supplementary Fig. 1b ). Reduced night-time sleep was mainly due to shortened sleeping bouts (Supplementary Fig. 1c ). To measure sleep quality and strength [57] , we analyzed the consolidation index (CI), the sleep latency, and the wake after sleep onset (WASO) index. Cyfip 85.1/+ flies revealed a sleep fragmentation phenotype and low sleep quality (Fig. 1c ) with an increased number of sleep bouts (Supplementary Fig. 1d ). The sleep latency and WASO (Supplementary Fig. 1e, f ) were increased in the Cyfip 85.1/+ mutants, suggesting an impairment in initiating and maintaining sleep. Fig. 1: CYFIP regulates the amount and quality of night-time sleep. a Representative sleep profile of control (black, n = 38) and Cyfip 85.1/+ (gray, n = 39) flies. Mean ± S.E.M. b , c Quantification of night sleep amount ( b ) and Consolidation Index (CI) at night ( c ) in control ( n = 75) and Cyfip 85.1/+ ( n = 75) flies. Two-tailed unpaired Student’s t test, **** p < 0.0001. Mean ± S.E.M. d Waking response after sleep perturbation at ZT16, ZT18 and ZT20 (marked by “*”) in control ( n = 24) and Cyfip 85.1 /+ ( n = 29) flies. Sleep loss is measured as the ratio between sleep after stimuli and the baseline sleep. Two-tailed unpaired Student’s t test, * p = 0.015. Mean ± S.E.M. e Sleep deprivation (12 h) and sleep profile of control ( n = 42) and Cyfip 85.1/+ ( n = 40) flies. Two-tailed unpaired Student’s t test, ****p < 0.0001. Mean ± S.E.M. Source data are provided as a Source Data file. Full size image Next, we probed the ability of flies to fall asleep after disturbing their sleep by external stimuli, following a previously described assay [58] , [59] . Flies were exposed to a light pulse of 5 min provided at ZT16, ZT18, and ZT20. The number of flies that were awakened by the light stimulus did not differ between Cyfip 85.1/+ and control conditions, because we chose a stimulus sufficiently strong to efficiently disturb the overall population (Supplementary Fig. 1g ). Notably, Cyfip mutants showed a reduction by approximately 50% of baseline sleep over the three time points, thus remaining awake for a longer time (Fig. 1d ), suggesting a state of increased arousal. The affected night-time sleep in the Cyfip heterozygous flies was not due to starvation, because food intake was not different between the two genotypes during daytime (Supplementary Fig. 1h ) nor 2 h before night onset (Supplementary Fig. 1i ). Although Cyfip expression during brain development has previously been described [39] , [56] , its pattern of expression in the adult brain has been less investigated. We created an HA-tagged fly (CYFIP N-HA ) using the CRISPR-Cas9 technology [60] (Supplementary Fig. 1j, k ) and observed an HA expression in the entire brain and at synapses, as shown by the colocalization with the synaptic protein Bruchpilot (Supplementary Fig. 1l ). To test whether the decrease in night sleep was caused by CYFIP depletion in the brain, we knocked-down Cyfip using two different UAS-Cyfip-RNAi lines (IR 1 and IR 2 ) driven by neuronal or glial promoters. We used the neuronal Ras2Gal4 driver, which is expressed largely in the overall neuronal population of adult fly CNS [61] , although not exclusively during larval development [62] , [63] , coupled with TubGal80 ts to specifically avoid lethal effects of Cyfip knockdown during larval development [56] . Cyfip RNAi driven by the Ras2Gal4;TubGal80 ts driver showed reduced Cyfip mRNA levels in adult fly heads (Supplementary Fig. 2a ) and caused a night-time sleep reduction, phenocopying both the sleep pattern and sleep deficits of Cyfip mutant flies (Supplementary Fig. 2b–g ). CYFIP abrogation in glia cells using RepoGal4 and NrvGal4 drivers did not affect night-time sleep (Supplementary Fig. 2h ), suggesting that the impaired Cyfip expression in neurons is mainly responsible for the observed sleep dysregulation. Since the Ras2Gal4 driver is not exclusively neuronal [62] , [63] , CYFIP might be required also in non-neuronal tissue to regulate night-time sleep behavior. We have previously shown that Cyfip reduction in GABAergic circuits causes social behavior abnormalities, an effect that is mediated by the mitochondrial transporter Aralar [43] . To investigate if Aralar or the involvement of the GABAergic system influence the sleep phenotype, we decreased Cyfip expression in GABAergic neurons and decreased excessive Aralar in the Cyfip 85.1/+ background. Under these experimental conditions, night-time sleep was not affected (Supplementary Fig. 3a, b ), and the Cyfip 85.1 / Aralar MI07552 flies maintained the sleep deficits (Supplementary Fig. 3b ), suggesting that social and sleep behaviors are regulated by Cyfip through two distinct pathways. Finally, abrogating CYFIP in a cluster of sleep-regulating neurons in the dorsal fan-shaped body (dFBs/ ExFl2 ) marked by the R23E10Gal4 driver [64] was sufficient to reduce the amount of night sleep (Supplementary Fig. 3c–d ). However, the involvement of other sleep-regulating circuits contributing to the sleep phenotype cannot be excluded. The sleep pattern results from a coordinated action of circadian and homeostatic mechanisms. To assess whether Cyfip 85.1/+ flies have circadian rhythm deficits, we tested flies in complete darkness (free running activity) and analyzed the periodicity. The two genetic conditions did not show any difference in circadian rhythm (Supplementary Fig. 3e–f ). In addition, no sleep defects were observed upon Cyfip RNAi expression in clock neurons or in pars intercerebralis or in ellipsoid body (Supplementary Fig. 3g ). Therefore, we examined whether reduced sleep in Cyfip mutants might arise from defective homeostatic regulation. Flies were mechanically sleep deprived (SD) at night for 12 h and sleep recovery was analyzed the following day. Cyfip 85.1/+ flies showed decreased daytime sleep and recovered less from sleep deprivation (Fig. 1e ). Similar results were obtained when Cyfip 85.1/+ were sleep deprived for 6 h and sleep recovery was measured in the following 6 h (Δ sleep) (Supplementary Fig. 3h ). Notably, Cyfip mutants exhibited reduced sleep rebound compared to control flies. Together, these findings suggest that Cyfip mutant flies exhibit reduced night-time sleep, suggesting an alteration in the homeostatic control of sleep due to deficits in sleep initiation and maintenance. Furthermore, Cyfip heterozygous flies show reduced sleep rebound after sleep deprivation, underlying deficits in sleep homeostatic mechanisms. Cyfip mutant flies have an imbalance in the NADP + /NADPH ratio Recently, it was shown that the sleep-promoting dorsal fan-shaped body neurons are sensitive to the balance of the intracellular NADP + /NADPH pool [18] . The activity of voltage-gated potassium channels of the Shaker-Hyperkinetic family (K v channels), important for neuronal excitability, is also inhibited by binding of the metabolite NADPH and therefore by low NADP + /NADPH ratios [65] . Shaker activity promotes the sleep state [18] , implying that low NADP + /NADPH ratios decrease sleep pressure. Given the observed alteration in homeostatic sleep control in Cyfip 85.1/+ mutant flies, we hypothesized that this might reflect an imbalance in brain NADP + /NADPH ratio oscillations in relevant time periods such as sleep initiation. We next measured the NADP + /NADPH ratio over the 24-h cycle in control and Cyfip 85.1 /+ flies using hydrophilic interaction chromatography coupled to targeted mass spectrometry analysis (HILIC-MS/MS). Importantly, we observed that in control flies the NADP + /NADPH ratio follows the behavioral state of the fly, i.e., rising at periods when the flies are awake and show increased locomotion activity (ZT0 and ZT12) and descending at ZT16 when sleep need is gradually reduced (Fig. 2a ). In contrast, Cyfip mutant flies do not show significant changes in the NADP + /NADPH ratio (between ZT8 and ZT16) or at the evening peak of locomotion activity (ZT12) (Fig. 2a ). Fig. 2: Cyfip mutant flies have an imbalance in the NADP + /NADPH ratio. a Upper inset, schematic of the experimental design; lower inset, quantification of the NADP + /NADPH ratio by HILIC-MS/MS in control and Cyfip 85.1/+ fly heads. Control n = 5, Cyfip 85.1/+ n = 5 over 24 h. n = independent samples, pool of 50 fly heads, for each time point. Two-way ANOVA followed by Tukey’s multiple comparisons test; time point effect p < 0.0001, genotype effect p < 0.0001, interaction effect p < 0.0001, F (6, 56) = 9.061, control ZT8 vs. ZT12 *** p = 0.0009; control ZT12 vs. ZT16 **p = 0.0022; Cyfip 85.1/+ ZT8 vs. Cyfip 85.1/+ ZT12 p = 0.99; Cyfip 85.1/+ ZT12 vs. Cyfip 85.1/+ ZT16 p = 0.34; Cyfip 85.1/+ ZT8 vs. Cyfip 85.1/+ ZT16 p = 0.74. Mean ± S.E.M. (see also Supplementary Data 6 ). Created with BioRender.com. b Upper inset, schematic of the experimental design. no-SD: undisturbed sleep, SD: sleep deprived. Lower inset, NADP + /NADPH ratio in control and Cyfip 85.1/+ fly heads in no-SD (control, n = 6, and Cyfip 85.1/+ , n = 6) and SD conditions (control, n = 6, and Cyfip 85.1/+ , n = 6). n = independent samples, pool of 23 fly heads. Two-way ANOVA followed by Sidak’s multiple comparisons test, sleep condition effect p = 0.0217, genotype effect p = 0.0243, interaction effect p = 0.022, F (1, 20) = 6.165, control no-SD vs. SD ** p = 0.0043; Cyfip 85.1/+ no-SD vs. SD p > 0.999, n.s. = not significant. Mean ± S.E.M. Source data are provided as a Source Data file. Full size image To assess if the imbalance in NADP + /NADPH ratio could reflect a deficit in the homeostatic sleep mechanism and in the sleep pressure accumulation, we monitored the NADP + /NADPH in the whole brain, in control and Cyfip 85.1/+ flies during undisturbed sleep (no-SD) and after 8 h of sleep deprivation (SD), as described [13] (Fig. 2b , upper inset). After sleep deprivation, control flies show an increase in the NADP + /NADPH ratio, possibly consistent with an increase in sleep need, while no changes in the NADP + /NADPH ratio were observed in the Cyfip 85.1/+ flies (Fig. 2b , lower inset). These data suggest that the biochemical reactions regulating NADP balance are dysregulated in the Cyfip 85.1/+ brain at sleep onset, thus inhibiting the accumulation of NADP + , hence decreasing the need for sleep necessary for initiating the sleep behavior. CYFIP regulates energy metabolism To characterize the molecular mechanism underlying sleep need and amount, we performed a comparative RNA-Seq in Cyfip mutants and control fly heads at ZT16 (Fig. 3a ), the period when Cyfip mutants showed impaired sleep (Fig. 1a ). Principal component (PC) analysis revealed a segregation of the samples according to the genotype (PC1 representing 55.4% of the data variance, Fig. 3b ). 1303 genes were differentially expressed, with 730 being upregulated and 573 downregulated in the Cyfip mutants (Fig. 3c, d and Supplementary Data 1 ). KEGG pathway enrichment analysis on the dysregulated genes (Fig. 3e and Supplementary Data 2 ) highlighted energy metabolism, lipid metabolism, amino acid metabolism, metabolism of cofactors and vitamins, and carbohydrate metabolism pathways being significantly dysregulated, possibly linking metabolic status and sleep homeostasis. Fig. 3: The Cyfip mutant transcriptome revealed a dysregulation of energy metabolism. a Schematic of the experimental design. Listed is the number of genes that were identified and passed consecutive filters. Created with BioRender.com. b Principal component analysis of RNA-seq data. Samples are color-coded according to the genotype. n = 3, where n = independent samples, pool of 20 fly heads. c Volcano plot showing the global transcriptional changes in control vs Cyfip 85.1/+ determined by RNA-seq. Moderated t test followed by the Benjamini-Hochberg method test for false discovery rate (FDR). Each circle represents one RNA, and colored circles represent differentially expressed genes (DEGs) significantly upregulated (FDR ≤ 0.05 and LFC ≥ 0.585 (in orange)) or significantly downregulated (FDR ≤ 0.05 and LFC ≤ −0.585 (in blue)). d Heatmap representing the DEGs significantly dysregulated in the different samples. e KEGG pathway enrichment analysis performed on the dysregulated mRNAs in Cyfip 85.1/+ mutants. Only the top interesting pathways for sleep and circadian rhythm behavior are represented in the scheme (see also Supplementary Data 2 ). Over-representation analysis (ORA) followed by Benjamini–Hochberg for false discovery rate. Parent KEGG terms are indicated in color. f Upregulated and downregulated genes (FDR ≤ 0.05, |LFC| ≥ 0.585) in Cyfip 85.1 /+ flies have been compared with the database for Drosophila wakefulness genes [13] . p = 4.514 −08 assessed by hypergeometric test, overlap between wakefulness-promoting genes and upregulated genes in Cyfip 85.1 /+ flies. Source data are provided in Supplementary Data files. Full size image To investigate whether the dysregulated genes in Cyfip 85.1/+ might affect sleep and wakefulness, we compared the identified upregulated and downregulated genes with a Drosophila database for genes associated with wakefulness and sleep state [13] . The upregulated genes in Cyfip 85.1/+ significantly overlapped with wakefulness-associated genes (27 out of 121, hypergeometric test p = 4.515 −08 ), as did 4 downregulated genes (Fig. 3f and Supplementary Data 3 ). The overlapping genes are related to oxidative stress and antioxidants (i.e. , GstE1 , and Cytochrome P450 subunits ), cellular metabolism, and immune response activity (i.e. , CG16756 ). Interestingly, around 25% of these genes (7 out of 27) are related to lipid metabolism. Among them, genes such as the fatty acid synthetase 1 ( FASN1 ) and Acetyl Coenzyme A synthase ( AcCoAS) are more involved in the fatty acid synthesis, while the malic enzyme ( Men ) supplies molecules for lipid synthesis (i.e., NADPH). In Drosophila , the malic enzyme ( Men ) is one of the main contributors to the NADPH pool for fatty acid biosynthesis [66] , [67] , together with the glucose-6-phosphate dehydrogenase ( Zw ) and the phosphogluconate dehydrogenase ( Pgd ) of the pentose phosphate pathway (PPP) and the cytosolic isocitrate dehydrogenase (IDH). We did not observe differential expression of IDH and the genes involved in the PPP, Zw , and Pgd , but we observed an over-expression of Men levels (Supplementary Data 1 ). Together, these results show that the wakeful behavior exhibited by Cyfip 85.1/+ during the night-time (ZT16) is associated with a transcriptome profile linked to wakefulness, pointing to a specific dysregulation of genes related to lipid homeostasis and to a possible role in the regulation of the NADP + /NADPH ratio. SREBP activity regulates the amount of night-time sleep The expression of genes related to lipid homeostasis (i.e., Men, FASN1 , acetyl-CoA carboxylase ( ACC )) is under the control of the sterol regulatory element-binding proteins (SREBPs). This regulation is conserved between flies and mammals [55] , [68] . To address whether dysregulation in SREBP expression and/or activity might be causative of the dysregulation of lipid genes, and in particular of Men , observed in Cyfip mutants, we compared the RNA-Seq dataset with transcriptomic datasets performed in human, murine, and Drosophila models overexpressing SREBP [69] , [70] , [71] . We identified 130 overlapping genes (Fig. 4a and Supplementary Data 4 ) and protein-protein interaction (PPI) network analysis revealed a major involvement in lipid metabolism, neuronal signaling, and protein synthesis (Supplementary Fig. 4a ). Subsequently, we compared the SREBP-overexpression dataset to genes associated with wakefulness and sleep [13] and found 21 common genes (Supplementary Data 5 ). Among those genes, 10 were identified as wakefulness-associated genes and dysregulated in Cyfip 85.1/+ flies, underlying the relevance of CYFIP and SREBP in such a regulation (hypergeometric test p = 3.467 −21 , Fig. 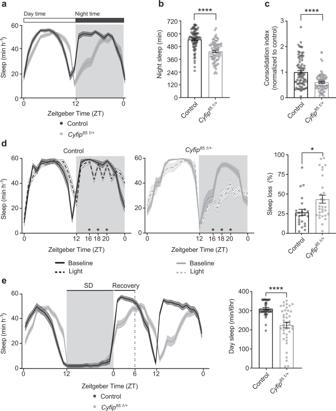Fig. 1: CYFIP regulates the amount and quality of night-time sleep. aRepresentative sleep profile of control (black,n= 38) andCyfip85.1/+(gray,n= 39) flies. Mean ± S.E.M.b,cQuantification of night sleep amount (b) and Consolidation Index (CI) at night (c) in control (n= 75) andCyfip85.1/+(n= 75) flies. Two-tailed unpaired Student’sttest, ****p< 0.0001. Mean ± S.E.M.dWaking response after sleep perturbation at ZT16, ZT18 and ZT20 (marked by “*”) in control (n= 24) andCyfip85.1/+(n= 29) flies. Sleep loss is measured as the ratio between sleep after stimuli and the baseline sleep. Two-tailed unpaired Student’sttest, *p= 0.015. Mean ± S.E.M.eSleep deprivation (12 h) and sleep profile of control (n= 42) andCyfip85.1/+(n= 40) flies. Two-tailed unpaired Student’sttest,****p< 0.0001. Mean ± S.E.M. Source data are provided as a Source Data file. 4b and Supplementary Table 1 ). Of those, AcCoAS, CG33110, Dbi, FASN1 and Men are directly involved in lipid metabolism. The overexpression of AcCoAS, FASN1 , and Men , in addition to other dysregulated wakefulness-associated genes, was confirmed by RT-qPCR (Fig. 4c ). These mRNAs are also found in databases containing gene expression profiles upon SREBP modulation [69] , [70] , [71] , further reinforcing their dependence on SREBP levels. Fig. 4: Increased lipid synthesis in Cyfip 85.1/+ is due to the upregulation of SREBP activity. Venn diagram showing ( a ) the overlap between the DEGs in Cyfip 85.1/+ and DEGs in SREBP-OE [69] , [70] , [71] . p = 0.98, ( b ) the overlap between the wakefulness-associated genes (WAGs) differentially expressed in Cyfip 85.1/+ and in SREBP-OE . p = 3.467 −21 , ( a–b ) one-sided hypergeometric test. c RT-qPCR in control and Cyfip 85.1 /+ flies at ZT16 normalized to rpl32 and rpl13 mRNA. FASN1 ** p = 0.007, FASN3 ** p = 0.0023, ACC * p = 0.0123, Lsd-1 * p = 0.0167, AcCoAS *** p = 0.0006, Men ** p = 0.0089, control and Cyfip 85.1 /+ ( n = 4). ATPCL * p = 0.0127, control ( n = 4) and Cyfip 85.1 /+ ( n = 3), n = pool of 15 fly heads. Mean ± S.E.M. d Representative blots and quantification of precursor and active SREBP, in controls and Cyfip 85.1/+ , between ZT12-ZT16, normalized over syntaxin and coomassie. SREBP-p, **** p < 0.0001 (control and Cyfip 85.1/+ , n = 20), SREBP-c, **p = 0.0029. Control ( n = 19) and Cyfip 85.1/+ ( n = 20), pool of 15 fly heads. Mean ± S.E.M. e Schematics of the Gal4-SREBP::GFP reporter and its activation. f GFP relative intensity, in control ( n = 12) and Cyfip 85.1 /+ ( n = 23) brains. ** p = 0.0017. Mean ± S.E.M. Scale bar = 50 µm. Maximum intensity Z-projections and magnification of the region marked by the square. g Night sleep in Ras2Gal4;TubGal80 ts/+ ( n = 20), UAS-Srebp wt/+ ( n = 19), UAS-Srebp c.del/+ ( n = 19), Ras2Gal4;TubGal80 ts > UAS-Srebp wt ( n = 24) and Ras2Gal4;TubGal80 ts > UAS-Srebp c.del ( n = 24) flies. One-way ANOVA and Sidak’s multiple comparisons test, **** p < 0.0001. Mean ± S.E.M. h Night sleep in controls ( n = 29), Cyfip 85.1 /+ ( n = 36) and Cyfip 85.1 / Srebp 189 ( n = 32) flies. Kruskal–Wallis and Dunn’s multiple comparisons test, **** p < 0.0001. Mean ± S.E.M. i Sleep rebound after 6 h of SD in controls ( n = 30), Cyfip 85.1 /+ ( n = 25) and Cyfip 85.1 / Srebp 189 ( n = 32). One-way ANOVA, Sidak’s multiple comparisons test; control vs. Cyfip 85.1 /+ * p = 0.019; Cyfip 85.1 /+ vs. Cyfip 85.1 / Srebp 189 * p = 0.027. Mean ± S.E.M. j Night sleep in control ( n = 20) and Cyfip 85.1 /+ ( n = 25) vehicle vs. control ( n = 17) and Cyfip 85.1 /+ ( n = 25) betulin treated flies. Two-way ANOVA and Tukey’s test, genotype-treatment interaction p < 0.0001, F (1, 83) = 18.25; **** p < 0.0001. Mean ± S.E.M. Two-tailed unpaired Student’s t test in ( c , d and f ). h , i n.s. = not significant. Source data are provided as a Source Data file. Full size image Next, we assessed whether SREBP levels and/or activity were altered in Cyfip 85.1 /+ flies. Notably, Cyfip 85.1 /+ mutant brain exhibited increased levels of precursor (SREBP-p) and active cleaved SREBP (SREBP-c) [72] , [73] compared to controls (Fig. 4d ) between ZT12 and ZT16. The increased SREBP activity in Cyfip 85.1/+ was further confirmed using a reporter for SREBP activation (Gal4-SREBP::GFP) [74] (Fig. 4e, f ). Together these results indicate that SREBP is overexpressed and overactive in Cyfip 85.1/+ mutant brain and suggest that SREBP might play a key role in sleep regulation, a function so far completely unexplored. We therefore directly assessed the consequences of increased SREBP activity on the Drosophila night-time sleep behavior. Neuronal overexpression (driven by Ras2Gal4 [62] ) of the full-length SREBP ( Srebp w t ) phenocopied the night-time sleep deficits observed in the Cyfip 85.1/+ , as well as upon Cyfip RNAi (Fig. 4g and Supplementary Fig. 4b ). Furthermore, upon constitutively active nuclear form of SREBP ( Srebp C.del ) overexpression, the amount of night sleep was decreased (Fig. 4g and Supplementary Fig. 4b ). Increased activity of SREBP had also an effect on the daytime sleep and the WASO index, namely the sleep quality (Supplementary Fig. 4c, d ). Thus, increased levels and/or activity of SREBP in neurons affect sleep behavior in flies, leading to the exacerbation of an insomnia-like phenotype. Notably, these data link SREBP to sleep behavior. To explore whether the increase in SREBP mediates the sleep disturbances in Cyfip mutant flies, we evaluated sleep in Cyfip 85.1 flies crossed with Srebp loss-of-function mutants ( Srebp 189/+ ) [75] . Cyfip 85.1 /Srebp 189 flies showed a restoration of the amount of night-time sleep (Fig. 4h and Supplementary Fig. 4e ), improved sleep quality (Supplementary Fig. 4f, g ) and sleep rebound after sleep deprivation (Fig. 4i ) while no effect on day sleep was observed. Furthermore, pharmacological reduction of SREBP activity using betulin (1 mM for 48 h), an inhibitor of SREBP activation [76] , also increased the night-time sleep in Cyfip mutants compared to untreated flies (Fig. 4j and Supplementary Fig. 5a, b ). Note that vehicle (DMSO in blue food) exacerbates sleep deficits (Supplementary Fig. 5b ). Importantly, such a treatment with betulin did not have any genotype-specific effect on food consumption (Supplementary Fig. 5c ). The pharmacological and genetic dampening of SREBP activity in Cyfip 85.1 flies reveals that SREBP modulation is relevant for proper night-time sleep amount and quality, and that increases in SREBP levels underlie the sleep disturbances seen in Cyfip 85.1 flies. The SREBP—Malic enzyme axis affects sleep Thus far, we have demonstrated a role for SREBP in sleep homeostasis in flies, and that NADP + /NADPH ratio oscillations  are altered in Cyfip 85.1/+ flies. HILIC-MS/MS revealed that the Cyfip 85.1 /Srebp 189 double mutant partially restored the NADP + /NADPH ratio at night-time onset (ZT12) (Fig. 5a ). As SREBP controls Men levels [77] , [78] and Men is a key contributor to the NADPH pool [66] , [67] , we hypothesized that the SREBP effects on sleep in Cyfip 85.1/+ might occur via Men -mediated regulation of the NADP + /NADPH. Wild-type flies undergoing sleep deprivation showed an increased Men mRNA expression (Supplementary Fig. 5d ), in agreement with previous observations [13] . No difference in Cyfip or Srebp mRNA expression was observed (Supplementary Fig. 5e, f ). Of note genetic reduction of Men in Cyfip 85.1 /+ flies ( Cyfip 85.1 /Men BG02790 ) was able to enhance the NADP + /NADPH ratio at control levels at night-time onset (Fig. 5a ). Consistently, we observed increased Men activity in Cyfip 85.1 /+ brains compared to controls at ZT10, before the night-time onset and Men activity was increased to control levels in the Cyfip 85.1 /Srebp 189 mutants (Fig. 5b ). Finally, when Men activity is genetically reduced in the Cyfip 85.1 /+ flies, loss of night-time sleep is ameliorated (Fig. 5c and Supplementary Fig. 5g ). Fig. 5: Men enzyme activity pairs SREBP to sleep. a NADP + /NADPH ratio at ZT12 by HILIC-MS/MS in control ( n = 10), Cyfip 85.1 /+ ( n = 10), Cyfip 85.1 / Srebp 189 ( n = 5), Srebp 189/+ ( n = 5) , Cyfip 85.1 / Men BG02790 ( n = 5) , Men BG02790+ ( n = 5). n = independent samples, pool of 45 fly heads. One-way ANOVA test and Sidak’s multiple comparisons test, control vs. Cyfip 85.1 /+ * p = 0.0359; Cyfip 85.1 /+ vs. Cyfip 85.1 / Men BG0279 * p = 0.0188; Cyfip 85.1 / Men BG02790 vs . Men BG02790 ** p = 0.0075; control vs. Men BG02790+ *** p = 0.0001. Mean ± S.E.M. b Men activity at ZT10, in control ( n = 5), Cyfip 85.1 /+ ( n = 6) and Cyfip 85.1 / Srebp 189 ( n = 6). n = independent samples, pool of 10 fly heads. Two-way repeated measures ANOVA and Tukey’s multiple comparisons test, time effect **** p < 0.0001, genotype effect *p = 0.0137, interaction **** p < 0.0001, F (138, 966) = 11.14; control vs. Cyfip 85.1 /+ * p = 0.0304; Cyfip 85.1 /+ vs. Cyfip 85.1 / Srebp 189 ** p = 0.0026; control vs. Cyfip 85.1 / Srebp 189 p = 0.57, n.s. = not significant. Mean ± S.E.M. c Quantification of night-time sleep in control ( n = 71), Cyfip 85.1 /+ ( n = 51), Cyfip 85.1 / Men BG02790 ( n = 60) and Men BG02790/+ ( n = 35) flies. One-way ANOVA and Sidak’s multiple comparisons test, control vs. Men BG02790/+ * p = 0.046; Cyfip 85.1 /+ vs. Cyfip 85.1 / Men BG0279 *** p = 0.0007; control vs. Cyfip 85.1 / Men BG0279 ** p = 0.0031; control vs. Cyfip 85.1/+ and Cyfip 85.1 / Men BG0279 vs. Men BG02790/+ **** p < 0.0001. Mean ± S.E.M. Source data are provided as a Source Data file. d Model. Full size image Interestingly, Men BG02790/+ flies showed an increase in night sleep amount and in the NADP + /NADPH ratio at night-time onset (Fig. 5a, c and Supplementary Fig. 5g ), demonstrating the property of Men to affect NADP levels and sleep behavior. Notably, despite the increase in Men transcript upon sleep deprivation in control flies, we did not observe changes in Men activity (Supplementary Fig. 5h ). On the contrary Men activity was increased, upon sleep deprivation, in Cyfip heterozygous flies (Supplementary Fig. 5i ). This is in line with the previously observed deficits in the NADP + /NADPH ratio after sleep deprivation in Cyfip 85.1/+ flies (Fig. 2b ) and further underlines that the pathological upregulation of Men drives changes in the NADP + /NADPH ratio and sleep deficits of Cyfip heterozygous flies. Altogether, these results demonstrate that the observed sleep deficits in the Cyfip 85.1/+ flies are mediated by the SREBP-Men-NADPH axis and show that SREBP activity and NADPH balance set the level of sleep amount at sleep onset. Using a Drosophila model for the human CYFIP1 haploinsufficiency ( Cyfip 85.1/+ mutant flies) a hotspot genetic variant increasing the risk for SCZ and a candidate risk factor for ASD, we describe a not yet identified molecular mechanism for sleep disturbances. Our findings uncover four key aspects in the regulation of sleep: (1) SREBP levels are altered in Cyfip mutant flies; (2) SREBP activity on wakefulness genes such as malic enzyme regulates night-time sleep onset and amount; (3) the NADP + /NADPH are regulated by the SREBP/Men axis ; (4) specific modulations of this metabolic pathway ameliorate the observed sleep deficits (Figs. 4 , 5 ) suggesting this pathway could be explored for the development of sleep disorder treatments. Specifically, our data show that increased activity of the sterol regulatory element-binding protein (SREBP) due to Cyfip heterozygosity (Fig. 4 ) induces an imbalance of the NADP + /NADPH ratio in the brain specifically at night, mediated by the overactivity of the malic enzyme (Fig. 5 ), resulting in deficits in sleep onset and amount (Fig. 1 and model in Fig. 5d ). Notably, night-time and daytime sleep features differ in flies [79] . Brain activity, measured as local field potential (LFP) and responsiveness to stimuli during night compared to daytime sleep, suggest different levels of homeostatic pressure on these processes throughout the 24 h [80] , [81] . While these differences have been reported, the function of daytime and night-time sleep in Drosophila remains unclear, although some hypotheses point to memory consolidation and synaptic homeostasis [80] , [81] . Therefore, the identification of factors, such as CYFIP, regulating differentially daytime and night-time sleep helps to shed light on the characteristics of these temporally distanced sleep. Only few genetic factors and mechanisms have been so far identified as regulators of daytime and night-time sleep, for instance, hormones, immune response, oxidative stress, and lipid binding molecules [79] . Here we show that at night-time Cyfip 85.1/+ flies revealed a dysregulation in transcripts regulating carbohydrate metabolism, monooxygenases ( i.e ., cytochrome P450), retinol, and lipid and energy metabolism among others, suggesting a convergence towards metabolic processes (Fig. 3 ). Of note, in a previous study, using unbiased proteomics in Cyfip 85.1/+ fly brain, we detected an upregulation of the ATP-Citrate Lyase, mitochondrial Men and Fatty-Acid Binding Protein (FABP) [43] , strengthening a role for CYFIP in metabolic regulation. Sleep restriction and sleep deprivation affect lipid gene expression and lipid profiles in murine and humans, supporting the idea that lipid synthesis and remodeling are relevant during sleep to restore the metabolic pool used during wakefulness supporting the organism physiology and neuronal activity [82] , [83] , [84] , [85] , [86] . We propose that increased expression of genes involved in energy metabolism and lipid synthesis in the Cyfip mutant reduces the homeostatic pressure at the night onset affecting the homeostatic sleep regulation (Fig. 5d ). SREBP is a central regulator of lipid biosynthesis and remodeling in many cell types [54] . SREBP functions have been studied primarily in lipogenic tissues (i.e., liver and adipose tissue) [87] , but have remained largely unexplored in the brain. Because the blood-brain barrier limits the transport of lipids in the brain, de novo synthesis of lipids in brain tissue is essential, and such a mechanism might require a specific regulatory process during wakefulness and sleep. Lipid homeostasis is essential for brain [88] , neuronal outgrowth [73] , [89] , [90] , myelination [91] , signaling, and energy supply [92] , [93] . Only recently, SREBP was shown to regulate lipid membrane biosynthesis, neuronal progenitor development [94] , synaptic genes expression, vesicle pool recycling, dendrite growth and development [73] , [90] and membrane function [69] . Here we show that modulation of SREBP is relevant to set the proper night-time sleep (Fig. 4 ) and that SREBP activity influences sleep onset through the modulation of the NADP + /NADPH level. It was recently discovered that the binding of NADP + or NADPH to the Shaker Kv channel complex and its β-subunit Hyperkinetic can inactivate or activate Kv currents regulating neuronal excitability [95] . Thus, the NADP + /NADPH ratio in specific sleep-inducing circuits (i.e., ExFl2 ) reflects neurons’ sleep pressure; when the NADPH cofactor is bound to Shaker, its activity is inhibited and wakefulness promoted, while the sleep switch is promoted by NADP + binding [18] . Our data show that over 24 h the NADP + /NADPH ratio in the whole brain increases at moments of intense locomotion/wakefulness and/or after sleep deprivation and decreases when sleep behavior is more solid with the reduction of sleep need. NADP fluctuations are therefore relevant to promote the night-time sleep onset, through its effect on sleep-promoting neuronal circuits. The accumulation of the NADP + over NADPH during sleep deprivation in wild-type flies, suggests its involvement in the homeostatic sleep regulation (Fig. 2 ). We cannot exclude that NADP + /NADPH changes might be related to increased locomotor activity: periods of motor/wakefulness increase sleep need. However, in support of our model, a mutation that impacts the NADP + /NADPH ratio alters sleep behavior (Fig. 5 ). Here, we propose that the driving force of the sleep deficits in Cyfip mutants is the dysregulation of the NADP +/ NADPH ratio (Fig. 2 ). Consistently, in Cyfip heterozygous flies, SREBP-driven over-expression and over-activity of the malic enzyme induce a reduced accumulation of NADP + at ZT12, possibly maintaining the sleep-regulating circuit OFF (Kv channels inhibited) and explaining the prolonged wakefulness at night-time onset (Fig. 5d ). Notably, a key player in regulating the NADP + /NADPH balance is the malic enzyme, which catalyzes the conversion of cytosolic malate to pyruvate, reducing NADP + at NADPH. Men expression and activity is pathologically upregulated in Cyfip 85.1/+ flies, resulting in the impaired NADP + /NADPH and sleep. Like Men, dysregulation of other enzymes involved in NADP + /NADPH homeostasis might contribute to sleep disorders. Sleep-wake disorders can have a negative impact on cognition, social function, mood, and quality of life in people and exacerbate the behavioral deficits in people suffering from psychiatric disorders [26] . Mutations in the human CYFIP1 gene have been linked to neurobehavioral disturbances, epilepsy, and psychiatric problems, emerging as risk factor for ASD and SCZ. Cyfip mutant flies exhibited sleep onset problems and low sleep rebound, a sign of deficits in homeostatic sleep regulation (Fig. 1 ), a feature also recently reported in children with ASD [96] . In addition, Cyfip heterozygous flies exhibit impaired associative learning [30] , a hallmark of sleep loss [97] , [98] , [99] , [100] , suggesting that sleep disorders and/or chronic sleep deprivation might contribute and exacerbate the cognitive defects reported in Cyfip mutants. We demonstrate that SREBP over-activation mediates the sleep deficits in the Cyfip heterozygous flies. Interestingly, the KO mouse model for SREBP1c displays SCZ-like behaviors and GABAergic hypofunction [101] , also commonly found in ASD. In addition, genome-wide association studies [102] classified the human SREBF1 gene (homolog of the Drosophila Srebp ) as a risk factor for SCZ, and single nucleotide variants in the DNA binding sites recognized by SREBF1 are associated with ASD [103] . Finally, the human SREBF1 gene has also been associated with excessive daytime sleepiness (EDS), a symptom of chronic insufficient sleep [104] . SREBP-Men inducing NADP + /NADPH alterations might therefore represent a common mechanism conserved in flies and mammals that contribute to a wide range of neurodevelopmental and neuropsychiatric disorders, including ASD and SCZ. Remarkably, alterations in NADP + /NADPH levels are observed in plasma of children with ASD [105] . Fly stocks and genetics Flies were maintained on standard cornmeal fly food at 25 °C, 60–80% relative humidity, in a 12-h light/dark cycle. Flies were trained to 12 h light/dark condition since the larval stage. Males 5–7 days after eclosion were used for all the experiments. The fly line used as control is a wild-type Canton-S w 1118 (BDSC 3605). The following stocks were previously described and kindly provided: Cyfip 85.1 and UAS-Cyfip-IR 1 by A. Giangrande (IGBMC, France); Ras2Gal4;TubGal80 ts , NrvGal4 and Gad1Gal4 by E.M.C. Skoulakis (BSRC, Greece); R23E10Gal4 by G. Miesenböck (CNCB, United Kingdom). RepoGal4 by L. Neukomm (Unil, Switzerland); ClkGal4_4.1 M , Mai179Gal4 and CryGal4_39 by F. Rouyer (CNRS, France); APLGal4 (VT043924-GAL4) by A. Fiala (Univ. Göttingen, Germany). The following fly lines were obtained from the Bloomington Stock Center (BDSC): Srebp 189 (39396), GAL4-dSREBPg.K-B31:UAS-GFP (‘SREBP activation reporter line’, 39612), UAS-Srebp WT (8236), UAS-Srebp c.del (constitutively active Srebp , 8244), Men BG02790 (12824), Aralar MI07552 (43727), PdfGal4 (6900), c819Gal4 (30849), c767Gal4 (30848) and Herm3xP3-ECFP,alphatub-piggyBacK10_M6 (32070). The UAS-Cyfip-IR 2 (37908) line was obtained from the Vienna Drosophila Resource Center. All transgenic lines were either generated in the w 1118 background or backcrossed 6 times into the w 1118 background. Temperature-induced experiments were performed as follows: UAS-Cyfip-IR flies expressing Ras2Gal4;TubGal80 ts and respective controls were raised at 18 °C throughout development to avoid the lethal developmental effect described for CYFIP abrogation. The TubGal80 ts was induced at 29 °C, 3–5 days after eclosion, for 3 days, allowing a strong Gal4 induction. From day 4 onwards flies were assessed for sleep behavior at 29 °C or used for RNA extraction. To test the expected lack of expression of the UAS-Cyfip-IR construct in flies expressing TubGal80 ts at 18 °C, Ras2Gal4;TubGal80 ts > UAS-Cyfip-IR flies and respective controls were raised, maintained, and tested at 18 °C. For the behavioral experiments involving UAS-Srebp wt and UAS-Srebp c.del , Ras2Gal4;TubGal80 ts > UAS-Srebp wt or UAS-Srebp c.del and respective control flies were raised at 25 °C throughout development, maintained and tested 5 to 7 days after eclosion at 25 °C. CRISPR/Cas9 generation of the CYFIP-HA tag fly strain Scarless genome editing approach based on the PiggyBac transposon (PBac) [106] was used to generate the Drosophila CYFIP N-HA tag. pBS-DsRed-attp-Cyfip N term-HA wSL cloning (donor plasmid): the 2614 bp fragment spanning the Cyfip gene (CG4931) start codon was PCR amplified using genomic DNA from nos-Cas9 (BDSC 78781) as a template and specific primers (5′-GAGCTCGAGCACGCCTCCGGTGATAGTAC −3′ and 5′-ACATCTAGACGGCATCAGAGGGATTCTCC-3′). The amplified fragment was cloned into the pBS-SK vector using the XhoI/XbaI sites. The resulting plasmid was used to amplify the left and right homology arms by PCR with the following primers (5′- GAGCTCGAGCACGCCTCCGGTGATAGTAC-3′ and 5′-CAATATGATTATCTTTCTAGGGTTAAATTCTAACAAGGCGGGGC-3′; 5′-GAGAAGATTACGCTAGCCGACG-3′ and 5′-AGAACTAGTCGGCATCAGAGGGATTCTCC-3′). The HA tag assembled from the primers containing the HA sequence: (5′- GCAGACTATCTTTCTAGGGTTAACCATTTCGCGCTGCTGGAGCATGATAAGCAGCCCAGCATGTACCC-3′ and 5′-CGTCGGCTAGCGTAATCTTCTCgGTGGCGTAATCGGGCACATCGTAGGGGTACATGCTGGGCTGCTTA-3′). Note that a silent mutation (g) was introduced in the protospacer adjacent motif (PAM) sequence to prevent cutting by the Cas9. The 3xP3-DsRed marker cassette flanked by TTAA target sequences was amplified from the pHD-sfGFP-ScarlessDsRed plasmid (DGRC stock 1365, kindly provided by B. McCabe, EPFL) with primers (5′-TTAACCCTAGAAAGATAATCATATTG-3′ and 5′-TTAACCCTAGAAAGATAGTCTGCG-3′). The generated fragments ( 3xP3-DsRed , left and right homology arms, and HA tag) were assembled using the Gibson assembly cloning standard protocols (New England Biolabs) and cloned into the pBS-SK vector, generating the donor plasmid. pCFD3-dU6-Cyfip gRNA cloning (gRNA plasmid): a sgRNA, 5′-TGATAAGCAGCCCAGCATG-3′, was designed using a on-line tool ( https://www.crisprscan.org ), synthetized as double-stranded oligonucleotide (5′-GTCGTGATAAGCAGCCCAGCATGA-3′ and 5′-AAACTCATGCTGGGCTGCTTATCA-3′), and cloned into the pCFD3-dU6:3gRNA vector (Addgene 49411) [107] . Donor and gRNA plasmids were injected into nos-Cas9 (II Chr) (BDSC 78781) embryos ( BestGene Inc . transgenic service). CRISPR homology DNA repair (HDR) transformants were screened based on the DsRed expression. HDR-positive stocks were then crossed with the PBac-transposase expressing fly stock (BDSC 32070) to induce the DsRed cassette excision. The HA insertion at the N-terminus of the Cyfip gene was confirmed amplifying (by PCR) the region surrounding the HA insertion in CYFIP N-HA/+ flies (Supplementary Fig. 1j ). WB analysis detected the HA tag above 130 kDa, in agreement with the molecular weight of the recombinant HA-CYFIP (Supplementary Fig. 1k ). The CYFIP N-HA tag flies were backcrossed with the w 1118 strain. Sleep-Wake activity assays Sleep assays were performed as previously described [57] . 5-7-day-old male flies raised in light/dark (LD)-entrained cultures were individually placed in 65 × 5 mm glass tubes containing 5% sucrose and 2% agar. Experiments were performed in an incubator with 60% humidity. Light was turned on at Zeitgeber Time 0 (ZT0) and off at ZT12. Fly activity was recorded for at least 3 consecutive days using the Drosophila Activity Monitoring (DAM) system (Trikinetics, Inc.). Activity records were collected in 1 min bins and analyzed using a custom-written R script (code available at: https://github.com/adrianclo/dam3 ). Sleep was defined as 5 consecutive minutes of inactivity. The sleep parameters were calculated as follows: Night-time sleep, the amount of sleep between ZT12-ZT24; Day-time sleep, the amount of sleep between ZT0 and ZT12; Night-time sleep bout number and length, number, and length of sleep events between ZT12 and ZT24; Latency to sleep is defined as the amount of time to the first sleep episode following light off (ZT12); Wake After Sleep Onset (WASO) is defined as the amount of time the fly is active following the first sleep episode between ZT12 and ZT24; Consolidation Index (CI) results from summing the squares of all the sleep-bout lengths in minutes divided by the total amount of sleep between ZT12 and ZT24 [57] . For sleep deprivation experiments, baseline sleep was recorded for 3 nights and then the flies were subjected to a sleep deprivation protocol using the Vortexer Mounting Plate (Trikinetics, Inc.) on the Multi-Tube Vortexer (VWR-2500). Sleep deprivation was carried out with the following sets: shaking for 2 s, every 60 s with a randomized protocol for 6 h (ZT12-ZT18) or 12 h. For each fly the Δ sleep was calculated as the amount of night-time sleep between ZT18 and ZT24 after deprivation (rebound sleep) minus amount of night sleep between ZT18 and ZT24 of the day before the deprivation (baseline sleep) for each fly. For 12 h of sleep deprivation, only flies exhibiting > 70% sleep loss throughout the night were used for the analysis. Arousal was tested similarly to [58] , [59] . In brief, flies were kept for 4 days at 12-h light/dark cycle. On the fourth night, a light pulse of 5 min was delivered at ZT16, ZT18, and ZT20. To analyze the effects of sleep perturbation by light stimuli at night, we calculated the sleep loss, at ZT16, ZT18 and ZT20, as follows: 100% – (night-time sleep after arousal/baseline night-time sleep) expressed as %. Flies with at least 2% of sleep loss were included in the analysis. Analysis of the awakenings was performed as described [108] : “not-responding” are flies with no activity 5 min before and 5 min after the stimulus and “responding” are flies with no activity 5 min before the stimulus and activity 5 min after the stimulus. "Awake flies", those that were moving in the 5 min preceding the stimulus, were excluded from the analysis. To evaluate rhythmicity, flies trained in 12:12 LD conditions were recorded for 4–5 days in 12:12 LD and then for 10 days in DD conditions. Actograms and periodicity were analyzed using the FaasX software (Rouyer & Boudinot, CNRF) (v. 1.21) [109] . Double-plotted actograms of average group activity were generated using the following settings: Light Cycle: LD_2400; Filter: Off; Hash Density: 08; Light on: ZT0 (08:30); Light off ZT12 (20:30); Fly survival: through the entire experiment. The periodicity was calculated using the chi-square periodogram method on at least 5 days in DD conditions, using the following settings: power > 120 and width > 1.5 h. Immunohistochemistry Brain dissection of male flies was carried out as previously described [110] . Brains were dissected on ice-cold in 1X PBS for 30 min maximum, fixed in 4% formaldehyde for 20 min, and washed for 30 min with PBST (1X PBS and 0.3% Triton-X). Blocking was performed with 10% normal goat serum (Sigma, cat. G9023) for 1 h. Tissues were stained overnight with the following antibodies: anti-GFP (Invitrogen, cat. A-11122, RRID: AB_221569, 1:1000), anti-BRP (DHSB, clone nc82, RRID: AB_2314866, 1:1000), and anti-HA 11 epitope tag (BioLegend, clone 16B12, cat. 901501, RRID: AB_2801249, 1:1000). The following secondary antibodies conjugated with Alexa Fluor (Thermo Fisher Scientific) were used at 1:1000 for 2 h at RT: anti-rabbit IgG 488 (cat. A-11034, RRID: AB_2576217), anti-mouse IgG 488 (cat. A-11029, RRID: AB_2534088), anti-mouse IgG 546 (cat. A-11030, RRID: AB_2534089) and anti-mouse IgG 647 (cat. A-21236, RRID: AB_2535805). After washes, the brains were mounted on Mowiol 4–88 mounting medium and imaged with a Leica SP8 confocal microscope using a 40x NA 1.25 water immersion objective. Images were taken using the same confocal and laser intensity settings. For the experiments with the SREBP activation reporter line, brain dissections were performed at ZT12 and fluorescent intensity was analyzed using ImageJ software (NIH). Fluorescence intensity was analyzed based on the sum of the different Z-stack intensity projections quantifying a ROI of the same dimension in 3 brain areas with strong GFP expression (superior lateral protocerebrum; suboesophageal ganglion and the ventrolateral protocerebrum). To account for background intensity, a ROI of the same dimension outside the brain tissue was subtracted. Western blotting Total protein extracts were prepared from fly heads and homogenized in RIPA buffer (150 mM NaCl, 50 mM Tris HCl, 1% Triton-X, 1% NaDoc, 1 mM EDTA, 1:100 Protease Inhibitor Cocktail from Sigma, 1:10 Phospho-Stop from Roche). Protein extracts were quantified using the Pierce™ BCA Protein Assay Kit (ThermoFisher, cat. 23225), separated by 10% SDS-Bis-Acrylamide gels and analyzed by Western blotting. The 10 kDa to 180 kDa PAGEruler pre stained Protein Ladder (ThermoFisher, cat. 26616) was used. The following antibodies were used: anti-SREBP (BD Biosciences, cat. 557036, RRID: AB_384985, 1:1000), anti-Syntaxin (DHSB, clone 8c3, RRID: AB_528484, 1:2000) and anti-HA 11 epitope tag (BioLegend, clone 16B12, RRID: AB_2801249, 1:1000) overnight at 4 °C. Membranes were incubated with DyLight (ThermoScientific) anti-mouse secondary antibodies 680- (cat. 35519, RRID: AB_1965956) and DyLight 800- (cat. SA5-10176, RRID: AB_2556756) at 1:5000 for 1 h and acquired using the Odyssey Infrared Imaging System (Li-COR Bioscience). Total protein staining (Li-COR Bioscience) or Coomassie staining was used for quantification. Signal intensity of the bands was quantified using ImageQuant (GE Healthcare) and each protein of interest was normalized for syntaxin and total protein content. RNA isolation and quantitative real time-PCR Fly heads were quickly collected at the specific time point (ZT16) or during undisturbed sleep and after 8 h of sleep deprivation (no-SD and SD). Total RNA was extracted using Trizol Reagent (Gibco) according to the manufacturer’s instructions. cDNA was prepared using the Superscript III first strand synthesis kit (Invitrogen, cat. 18080093) and random primers (Promega). RT-qPCR was performed on the iCycler iQ Real-Time PCR Detection System (Bio-Rad Laboratories) using SYBR Green-based detection (Roche, cat. 04887352001). Transcript levels were determined from threshold cycle values based on a standard curve derived from serial cDNA dilutions. Relative mRNA expression levels were normalized to Rpl13 or Rpl32 using the comparative ΔΔCT method. 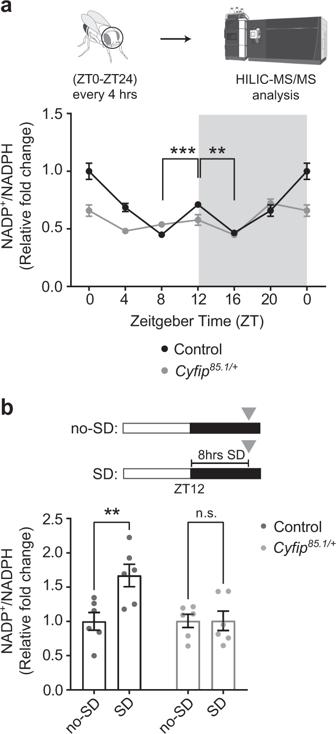Fig. 2:Cyfipmutant flies have an imbalance in the NADP+/NADPH ratio. aUpper inset, schematic of the experimental design; lower inset, quantification of the NADP+/NADPH ratio by HILIC-MS/MS in control andCyfip85.1/+fly heads. Controln= 5,Cyfip85.1/+n= 5 over 24 h.n= independent samples, pool of 50 fly heads, for each time point. Two-way ANOVA followed by Tukey’s multiple comparisons test; time point effectp< 0.0001, genotype effectp< 0.0001, interaction effectp< 0.0001,F(6, 56)= 9.061, control ZT8 vs. ZT12 ***p= 0.0009; control ZT12 vs. ZT16**p= 0.0022;Cyfip85.1/+ZT8 vs.Cyfip85.1/+ZT12p= 0.99;Cyfip85.1/+ZT12 vs.Cyfip85.1/+ZT16p= 0.34;Cyfip85.1/+ZT8 vs.Cyfip85.1/+ZT16p= 0.74. Mean ± S.E.M. (see also Supplementary Data6). Created with BioRender.com.bUpper inset, schematic of the experimental design. no-SD: undisturbed sleep, SD: sleep deprived. Lower inset, NADP+/NADPH ratio in control andCyfip85.1/+fly heads in no-SD (control,n= 6, andCyfip85.1/+,n= 6) and SD conditions (control,n= 6, andCyfip85.1/+,n= 6).n= independent samples, pool of 23 fly heads. Two-way ANOVA followed by Sidak’s multiple comparisons test, sleep condition effectp= 0.0217, genotype effectp= 0.0243, interaction effectp= 0.022,F(1, 20)= 6.165, control no-SD vs. SD **p= 0.0043;Cyfip85.1/+no-SD vs. SDp> 0.999, n.s. = not significant. Mean ± S.E.M. Source data are provided as a Source Data file. The primers used are listed in Supplementary Table 2 . 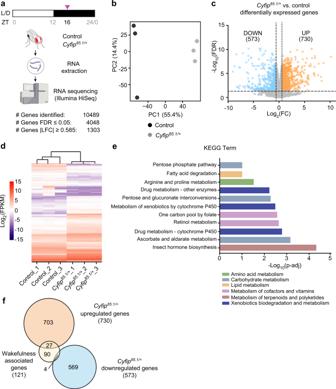Fig. 3: TheCyfipmutant transcriptome revealed a dysregulation of energy metabolism. aSchematic of the experimental design. Listed is the number of genes that were identified and passed consecutive filters. Created with BioRender.com.bPrincipal component analysis of RNA-seq data. Samples are color-coded according to the genotype.n= 3, wheren= independent samples, pool of 20 fly heads.cVolcano plot showing the global transcriptional changes in control vsCyfip85.1/+determined by RNA-seq. Moderatedttest followed by the Benjamini-Hochberg method test for false discovery rate (FDR). Each circle represents one RNA, and colored circles represent differentially expressed genes (DEGs) significantly upregulated (FDR ≤ 0.05 and LFC ≥ 0.585 (in orange)) or significantly downregulated (FDR ≤ 0.05 and LFC ≤ −0.585 (in blue)).dHeatmap representing the DEGs significantly dysregulated in the different samples.eKEGG pathway enrichment analysis performed on the dysregulated mRNAs inCyfip85.1/+mutants. Only the top interesting pathways for sleep and circadian rhythm behavior are represented in the scheme (see also Supplementary Data2). Over-representation analysis (ORA) followed by Benjamini–Hochberg for false discovery rate. Parent KEGG terms are indicated in color.fUpregulated and downregulated genes (FDR ≤ 0.05, |LFC| ≥ 0.585) inCyfip85.1/+flies have been compared with the database forDrosophilawakefulness genes13.p= 4.514−08assessed by hypergeometric test, overlap between wakefulness-promoting genes and upregulated genes inCyfip85.1/+flies. Source data are provided in Supplementary Data files. cDNA library generation and RNA-sequencing Fly heads were quickly collected at ZT16 using liquid nitrogen. Total RNA was isolated using Trizol Reagent (Gibco) according to the manufacturer’s instructions to extract total RNA. RNA quality was evaluated on a Fragment Analyzer (Agilent Technologies, Inc., Santa Clara, CA 95051, USA) and the RQN were between 8.5 and 9.7. RNA-seq libraries were prepared using 500 ng of total RNA and Illumina TruSeq Stranded mRNA reagents (Illumina; San Diego, California, USA) on a Sciclone liquid handling robot (PerkinElmer; Waltham, Massachusetts, USA) using a PerkinElmer-developed automated script. Cluster generation was performed with the resulting libraries using the Illumina HiSeq SR Cluster Kit v4 reagents and sequenced on the Illumina HiSeq 2500 using HiSeq SBS Kit v4 reagents. Sequencing data were demultiplexed using the bcl2fastq Conversion Software (v. 2.20, Illumina; San Diego, California, USA). RNA-sequencing data processing and analysis Purity-filtered reads were adapter- and quality trimmed with Cutadapt (v. 1.8) [111] . Reads matching to ribosomal RNA sequences were removed with fastq_screen (v. 0.9.3). Remaining reads were further filtered for low complexity with reaper (v. 15-065) [112] . Reads were aligned against Drosophila melanogaster BDGP6.86 genome using STAR (v. 2.5.2b) [112] and the estimation of the isoforms abundance was computed using RSEM (v. 1.2.31) [113] . The number of read counts per gene locus was summarized with htseq-count (v. 0.6.1) [114] using Drosophila melanogaster BDGP6.86 gene annotation. 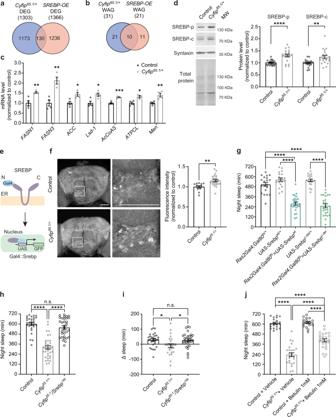Fig. 4: Increased lipid synthesis inCyfip85.1/+is due to the upregulation of SREBP activity. Venn diagram showing (a) the overlap between the DEGs inCyfip85.1/+and DEGs in SREBP-OE69,70,71.p= 0.98, (b) the overlap between the wakefulness-associated genes (WAGs) differentially expressed inCyfip85.1/+and inSREBP-OE.p= 3.467−21, (a–b) one-sided hypergeometric test.cRT-qPCR in control andCyfip85.1/+flies at ZT16 normalized torpl32andrpl13mRNA.FASN1**p= 0.007,FASN3**p= 0.0023,ACC*p= 0.0123,Lsd-1*p= 0.0167,AcCoAS***p= 0.0006,Men**p= 0.0089, control andCyfip85.1/+(n= 4).ATPCL*p= 0.0127, control (n= 4) andCyfip85.1/+(n= 3),n= pool of 15 fly heads. Mean ± S.E.M.dRepresentative blots and quantification of precursor and active SREBP, in controls andCyfip85.1/+, between ZT12-ZT16, normalized over syntaxin and coomassie. SREBP-p, ****p< 0.0001 (control andCyfip85.1/+,n= 20), SREBP-c,**p= 0.0029. Control (n= 19) andCyfip85.1/+(n= 20), pool of 15 fly heads. Mean ± S.E.M.eSchematics of theGal4-SREBP::GFPreporter and its activation.fGFP relative intensity, in control (n= 12) andCyfip85.1/+(n= 23) brains. **p= 0.0017. Mean ± S.E.M. Scale bar = 50 µm. Maximum intensity Z-projections and magnification of the region marked by the square.gNight sleep inRas2Gal4;TubGal80ts/+(n= 20),UAS-Srebpwt/+(n= 19),UAS-Srebpc.del/+(n= 19),Ras2Gal4;TubGal80ts>UAS-Srebpwt(n= 24) andRas2Gal4;TubGal80ts>UAS-Srebpc.del(n= 24) flies. One-way ANOVA and Sidak’s multiple comparisons test, ****p< 0.0001. Mean ± S.E.M.hNight sleep in controls (n= 29),Cyfip85.1/+(n= 36) andCyfip85.1/Srebp189(n= 32) flies. Kruskal–Wallis and Dunn’s multiple comparisons test, ****p< 0.0001. Mean ± S.E.M.iSleep rebound after 6 h of SD in controls (n= 30),Cyfip85.1/+(n= 25) andCyfip85.1/Srebp189(n= 32). One-way ANOVA, Sidak’s multiple comparisons test; control vs.Cyfip85.1/+*p= 0.019;Cyfip85.1/+vs.Cyfip85.1/Srebp189*p= 0.027. Mean ± S.E.M.jNight sleep in control (n= 20) andCyfip85.1/+(n= 25) vehicle vs. control (n= 17) andCyfip85.1/+(n= 25) betulin treated flies. Two-way ANOVA and Tukey’s test, genotype-treatment interactionp< 0.0001,F(1, 83)= 18.25; ****p< 0.0001. Mean ± S.E.M. Two-tailed unpaired Student’sttest in (c,dandf).h,in.s. = not significant. Source data are provided as a Source Data file. 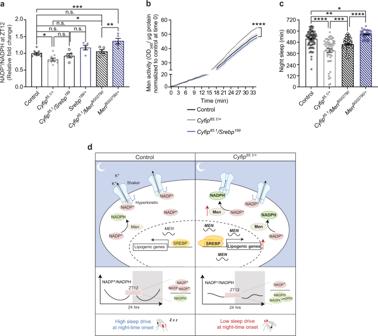Fig. 5: Men enzyme activity pairs SREBP to sleep. aNADP+/NADPH ratio at ZT12 by HILIC-MS/MS in control (n= 10),Cyfip85.1/+(n= 10),Cyfip85.1/Srebp189(n= 5),Srebp189/+(n= 5), Cyfip85.1/MenBG02790(n= 5), MenBG02790+(n= 5).n= independent samples, pool of 45 fly heads. One-way ANOVA test and Sidak’s multiple comparisons test, control vs.Cyfip85.1/+*p= 0.0359;Cyfip85.1/+vs.Cyfip85.1/MenBG0279*p= 0.0188;Cyfip85.1/MenBG02790vs. MenBG02790**p= 0.0075; control vs.MenBG02790+***p= 0.0001. Mean ± S.E.M.bMen activity at ZT10, in control (n= 5),Cyfip85.1/+(n= 6) andCyfip85.1/Srebp189(n= 6).n= independent samples, pool of 10 fly heads. Two-way repeated measures ANOVA and Tukey’s multiple comparisons test, time effect ****p< 0.0001, genotype effect*p= 0.0137, interaction ****p< 0.0001,F(138, 966)= 11.14; control vs.Cyfip85.1/+*p= 0.0304;Cyfip85.1/+vs.Cyfip85.1/Srebp189**p= 0.0026; control vs.Cyfip85.1/Srebp189p= 0.57, n.s. = not significant. Mean ± S.E.M.cQuantification of night-time sleep in control (n= 71),Cyfip85.1/+(n= 51),Cyfip85.1/MenBG02790(n= 60) andMenBG02790/+(n= 35) flies. One-way ANOVA and Sidak’s multiple comparisons test, control vs.MenBG02790/+*p= 0.046;Cyfip85.1/+vs.Cyfip85.1/MenBG0279***p= 0.0007; control vs.Cyfip85.1/MenBG0279**p= 0.0031; control vs.Cyfip85.1/+andCyfip85.1/MenBG0279vs.MenBG02790/+****p< 0.0001. Mean ± S.E.M. Source data are provided as a Source Data file.dModel. Quality of the RNA-Seq data alignment was assessed using RSeQC (v. 2.3.7) [115] . Statistical analysis was performed for genes in R (R v. 3.3.2). Genes with low counts were filtered according to the rule of 1 count per million (cpm) in at least 1 sample. Library sizes were scaled using TMM normalization (EdgeR package v. 3.14.0) [116] and log-transformed with the limma voom function (Limma package version 3.28.21) [117] . Differential expression was computed with limma [118] by fitting all samples into a linear model. Next the comparison between Cyfip 85.1/+ vs control was performed. Moderated t-test was used for each contrast. The adjusted p-value was computed by the Benjamini-Hochberg method, controlling for false discovery rate (FDR or adj. p -value). Genes with an adjusted p -value ≤ 0.05 (FDR ≤ 0.05) and log2 fold change greater than 0.585 or smaller than −0.585 (|LFC| ≥ 0.585, 50% fold increase/33% decrease) were considered differentially expressed (DEGs). KEGG pathways analysis for the DEGs was performed using GeneTrail2 3.0 ( https://genetrail2.bioinf.uni-sb.de ) [119] . Over-representation analysis (ORA) was applied with the Benjamini-Hochberg false discovery rate test. Hypergeometric test was performed using R ( https://stat.ethz.ch/R-manual/R-devel/library/stats/html/Hypergeometric.html ). Protein-protein interaction (PPI) network analysis Network analysis on the gene overlap between SREBP overexpression DEG databases and dysregulated Cyfip 85.1/+ genes at ZT16 was performed using the online bioinformatic tool STRING interactome ( https://string-db.org ) for PPI networks with a high confidence score cutoff and experimental evidence required. The PPI networks were graphed and visualized using Cytoscape 3 (RRID:SCR_003032). Metabolite extraction and protein quantification Drosophila heads (45–50) were extracted and homogenized adding 150 µL of MeOH:H 2 O (4:1), in the Precellys 24 sample Homogenizer (2 × 20 s at 10000 rpm, Bertin Technologies, Rockville, MD, US) with ceramic beads. The bead beater (Cryolys) was air-cooled down at a flow rate of 110 L/min at 6 bar. After centrifugation, the resulting supernatant was collected and transferred into LC vials for analysis. Protein pellets were evaporated and lysed in 20 mM Tris-HCl (pH 7.5), 4 M guanidine hydrochloride, 150 mM NaCl, 1 mM Na 2 EDTA, 1 mM EGTA, 1% Triton, 2.5 mM sodium pyrophosphate, 1 mM beta-glycerophosphate, 1 mM Na 3 VO 4 , 1 µg/ml leupeptin using the Cryolys Precellys 24 sample Homogenizer (2 × 20 s at 10000 rpm, Bertin Technologies, Rockville, MD, US) with ceramic beads. BCA Protein Assay Kit was used to measure total protein concentration. Hydrophilic interaction liquid chromatography coupled to tandem mass spectrometry (HILIC-MS/MS) analysis Extracted samples were analyzed by HILIC - MS/MS [120] , [121] in negative ionization mode using a 6495 triple quadrupole system (QqQ) interfaced with 1290 UHPLC system (Agilent Technologies). Chromatographic separation was carried out in a SeQuant ZIC-pHILIC (100 mm, 2.1 mm I.D. and 5 μm particle size, Merck, Damstadt, Germany) column. The mobile phase was composed of A = 20 mM ammonium acetate and 20 mM NH 4 OH in water at pH 9.7 and B = 100% ACN. The linear gradient elution from 90% (0–1.5 min) to 50% B (8–11 min) down to 45% B (12–15 min). Finally, the initial chromatographic conditions were established as a post-run during 9 min for column re-equilibration. The flow rate was 300 μL/min, column temperature at 30 °C and the sample injection volume was 2 µl. ESI source conditions were set as follows: dry gas temperature 290 °C and flow 14 L/min, sheath gas temperature 350 °C, nebulizer 45 psi, and flow 12 L/min, nozzle voltage 0 V, and capillary voltage −2000 V. Dynamic Multiple Reaction Monitoring (dMRM) was used as acquisition mode with a total cycle time of 600 ms. Optimized collision energies for each metabolite were applied. Pooled QC samples (representative of the entire sample set) were analyzed periodically (every 6 samples) throughout the overall analytical run in order to assess the quality of the data, correct the signal intensity drift (attenuation in most cases, that is inherent to LC-MS technique and MS detector due to sample interaction with the instrument over time) and remove the peaks with poor reproducibility (CV > 30%) [122] , [123] . In addition, a series of diluted quality controls (dQC) were prepared by dilution with methanol: 100% QC, 50%QC, 25%QC, 12.5%QC and 6.25%QC. Then, metabolites were selected also considering the linear response on the diluted QC series. Data processing Raw LC-MS/MS data were processed using the Agilent Quantitative analysis software (v. B.07.00, MassHunter Agilent technologies). Relative quantification of the metabolites was based on EIC (Extracted Ion Chromatogram) areas for the monitored MRM transitions. The obtained tables (containing peak areas of detected metabolites across all samples) were exported to R software and signal intensity drift correction and noise filtering (using CV (QC features) > 30%, if necessary) were compiled within the MRM PROBS software [124] . Drosophila betulin administration Betulin (Sigma, Cat. B9757) was dissolved in DMSO. The solution was added to the Formula 4–24® Instant Drosophila Medium (blue food) in water to a final concentration of 1 mM. Male flies 5-7 days old were placed in plastic vials containing the blue food with betulin or vehicle and fed ad libitum for 48 h. Vehicle treatment consisted of solvent (DMSO) added to blue food. Food intake assay A colorimetric estimation of food intake was performed as previously described [43] . To monitor food intake during the period ZT0-ZT12, groups of 5–7 days old male flies were transferred to food containing 2.5% (w/v) non-degradable dye (Erioglaucine blue disodium salt; Sigma-Aldrich, cat. 861146), 2% agar and 5% sucrose every 2 h from ZT0 to ZT12, left to feed ad libitum for 2 h then collected for food intake assessment. For betulin treatment, flies were transferred for 48 h on food containing 2.5% (w/v) erioglaucine blue, 2% agar and 5% sucrose added with water, DMSO, or 1 mM betulin dissolved in DMSO. After feeding period, individual flies were homogenized in 65 µl of chilled PBS 1X and centrifuged at 10.000 g for 1 min. Finally, 50 µl of supernatant was used for absorbance recording at 620 nm using a spectrophotometer. NADP + /NADPH quantification NADP + /NADPH ratio was measured from brain lysates using the NADP + /NADPH Quantification Colorimetric Kit (Abcam, cat. ab65349) following the manufacturer’s instructions. Colorimetric measurements were performed at 450 nm using a Hidex Sense 96-wells plate reader. 23 fly heads per sample were used. Malic enzyme assay Enzymatic activity of the malic enzyme was performed as previously described [67] . Briefly, 10 heads per sample from 5 day old male flies, at ZT10 or after 8 h of sleep deprivation (no-SD vs. SD), were homogenized in freshly prepared grinding buffer (100 mM Tris-HCl, 0.15 mM Na 2 NADP, pH 7.4) and centrifuged at 15000 g 4 °C for 5 min to pellet the debris. 10 µl of extract was used for total protein quantification. Activity assay was performed in a 96-well plate using 10 µl of extract and 100 µl of freshly prepared buffer (100 mM Tris-HCl, 0.34 mM Na 2 NADP, 50 mM MnCl 2 , 50 mM malate, pH 7.4). Absorbance was measured every 30 s for 20 min at OD 340, 25 °C using a Hidex Sense Spectrophotometer (Labgene). Samples were analyzed in technical duplicates. The  absorbance was normalized to the total protein content measured by the Pierce BCA Protein Assay Kit. Statistics Statistical analyses were carried out using Prism (v. 8.0) and/or R. The statistical tests are listed in the respective figure legends and in Supplementary Data 6 . The normal distribution of the data was assessed using the Shapiro-Wilk test prior to statistical analyses. For comparison between two independent groups, unpaired two-tailed Student’s t test or the Mann–Whitney test for non-parametric data were used. When comparing more than two independent groups, one-way analysis of variance (ANOVA) was used followed by Tukey’s or Holm Sidak’s multiple comparisons test or the non-parametric Kruskal–Wallis test followed by Dunn’s post hoc test correction for multiple comparisons. Two-way analysis of variance (ANOVA) followed by Tukey’s multiple comparisons test for non-repeated measurement data, two-way analysis of variance (ANOVA) with repeated measurement followed by Holm Sidak’s or Tukey’s post hoc test was used to examine two independent variables. Fisher’s exact test and hypergeometric distribution analyses were assessed using R. For all analyses, P -values < 0.05 were considered significant and annotated as follows: *p < 0.05, **p < 0.01, ***p < 0.001, ****p < 0.0001. Results are presented as mean ± standard error of the mean (S.E.M.). Exact P- values for *p < 0.05, **p < 0.01 and ***p < 0.001, n of independent samples, or individual flies, or pool of flies (see figure legends), and descriptive statistics are reported in Supplementary Data 6 . Reporting summary Further information on research design is available in the Nature Portfolio Reporting Summary linked to this article.